Glassiness and exotic entropy scaling induced by quantum fluctuations in a disorder-free frustrated magnet When spins are arranged in a lattice of triangular motif, the phenomenon of frustration leads to numerous energetically equivalent ground states, and results in exotic states such as spin liquid and spin ice. Here we report an alternative situation: a system, classically a liquid, freezes in the clean limit into a glassy state induced by quantum fluctuations. We call such glassy state a spin jam. The case in point is a frustrated magnet, where spins are arranged in a triangular network of bipyramids. Quantum corrections break the classical degeneracy into a set of aperiodic spin configurations forming local minima in a rugged energy landscape. This is established by mapping the problem into tiling with hexagonal tiles. The number of tessellations scales with the boundary length rather than its volume, showing the absence of local zero-energy modes. Low-temperature thermodynamics is discussed to compare it with other glassy materials. It is well known, since the classical work of Pauling on ice [1] , that certain systems can exhibit an extensive number of energetically equivalent ground states, leading to finite entropy at low temperatures [2] , [3] . In a spin ice, states are separated by local energy barriers, and the spins freeze into one of the equivalent states at low-enough temperatures [4] , [5] . In pyrochlore with large spins, locally confined zero-energy motions of spins are possible, which can lead to a classical spin liquid state [6] . When quantum effects are taken into account, for small spins, such systems may settle into a super-position of states, forming a quantum spin-liquid [5] , as suggested by Anderson [7] . A closely related but distinct type of systems is glassy systems. One example is amorphous alloys in which the atoms are arranged in a disordered way [8] , [9] . Another is spin glass systems in which low concentration of magnetic impurities interact via random long-range interactions [10] , [11] . In such systems, randomness (or quenching) is the driving force for the freezing phenomena. The randomness, however, makes it difficult to fully understand the complex physics of the freezing phenomenon. Interesting effective models for glassy behaviour without disorder have been presented to understand various types of glasses. For example, glassy behaviour has been explored in systems with long-range interactions [12] and in models with hard-core classical constraints and stochastic dynamics known as kinetically constrained models [13] , as well as in certain quantum plaquette and quantum dimer models [14] , [15] . Here we show that a glass state, a spin jam, can actually arise from simple nearest neighbour Heisenberg interactions with full O(3) rotational symmetry at low temperatures owing to quantum effects. Moreover, this behaviour may be present in real materials, and may provide a framework to understand the unconventional [16] glassy behaviours found in classes of frustrated magnets, such as SrCr 9 p Ga 12-9 p O 19 (SCGO( p )) [2] , [17] , [18] , [19] and qs-ferrites like Ba 2 Sn 2 ZnGa 3 Cr 7 O 22 (BSZGCO) [20] , with spin 3/2 that are highly crystalline and their glassiness seems to be insensitive to disorder [18] , [21] . Motivated by the seemingly intrinsic nature of the glassy behaviour in such crystalline spin glasses, we explore a Heisenberg model on a magnetic lattice realized in SCGO and qs-ferrites. The magnetic lattice of interest is a triangular network of bipyramids that are formed by two corner-sharing tetrahedra and are connected by linking triangles (see Fig. 1a and Supplementary Fig. 1 ). Here we study a simple nearest neighbour-spin interaction Hamiltonian . Classically, any spin configuration in which each tetrahedron and linking triangle has a total zero spin is a ground state. There are infinite number of energetically equivalent configurations. 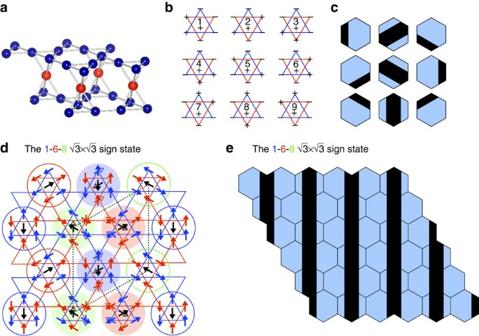Figure 1: The triangular network of bipyramids and its classical ground states. (a) The kagome-triangular-kagome tri-layer, forming the triangular network of bipyramids. Each bipyramid is composed of two corner-sharing tetrahedra. The blue and red spheres represent kagome and triangular sites, respectively. (b) The internally collinear states for each bipyramid are categorised by assigning for each spin a binary sign (representing a parallel (+) or antiparallel (−) direction relative to the colour). These states may be viewed as the 18 elements ofby first specifying the sign of the central spin, and specifying one spin in the upper and the lower layers of the bipyramid with the same sign. For visualisation, we simply label the first nine states numerically 1..9, and the counterpart (associated with flipping all the signs) as 10..18. (c) The hexagon tiles. The six corners of the hexagon tile represent the six spins forming the upper and the lower triangles of the bipyramid. The black and blue colours on the boundary represent (+) and (−) signs on the boundary, respectively. (d) Acollinear bipyramid spin state constructed from the combination of thelong-range ordered 1-6-8 sign state and aorder of the tri-colour (the red, blue, green represent the three spin directions of a 120oconfiguration). The unfilled arrows in the middle represent the spins in motion, and the colour-shadowed circles represent the affected bipyramids. Such spaghetti excitations can act as domain boundaries. (e) The 1-6-8 state as ind, but shown as a periodic tiling in the hexagon representation. Figure 1: The triangular network of bipyramids and its classical ground states. ( a ) The kagome-triangular-kagome tri-layer, forming the triangular network of bipyramids. Each bipyramid is composed of two corner-sharing tetrahedra. The blue and red spheres represent kagome and triangular sites, respectively. ( b ) The internally collinear states for each bipyramid are categorised by assigning for each spin a binary sign (representing a parallel (+) or antiparallel (−) direction relative to the colour). These states may be viewed as the 18 elements of by first specifying the sign of the central spin, and specifying one spin in the upper and the lower layers of the bipyramid with the same sign. For visualisation, we simply label the first nine states numerically 1..9, and the counterpart (associated with flipping all the signs) as 10..18. ( c ) The hexagon tiles. The six corners of the hexagon tile represent the six spins forming the upper and the lower triangles of the bipyramid. The black and blue colours on the boundary represent (+) and (−) signs on the boundary, respectively. ( d ) A collinear bipyramid spin state constructed from the combination of the long-range ordered 1-6-8 sign state and a order of the tri-colour (the red, blue, green represent the three spin directions of a 120 o configuration). The unfilled arrows in the middle represent the spins in motion, and the colour-shadowed circles represent the affected bipyramids. Such spaghetti excitations can act as domain boundaries. ( e ) The 1-6-8 state as in d , but shown as a periodic tiling in the hexagon representation. Full size image An important subset of these states is the set of states in which the spins in each bipyramid are collinear [22] . It is well established that collinear configurations are commonly favored in frustrated magnets [23] such as pyrochlore. The mechanism for such a selection is known as order from disorder [24] . In other examples, such as the Heisenberg kagome antiferromagnet, extensive analysis [25] , [26] were carried out showing the selection of planar spin configuration, whose close relation to SCGO has been also discussed there. Our lattice, on the other hand, contains both tetrahedra favoring collinearity as well as linking triangles preferring planar 120° configurations. Note, in passing, that in most cases with co-linear spin configurations the collinearity is global over the entire lattice, whereas here the collinear direction is not global. Henceforth, we will refer to such states simply as locally collinear (LC) states. We would also like to emphasise one of our main results is the identification of metastable states generated by the order-by-disorder mechanism, rather than the, perhaps more common, search for the global ground state. Our main results are the following. When taking into account the order-by-disorder quantum corrections, the classical degeneracy is broken into a set of local minima in a rugged energy landscape, which are separated by large energy barriers, over a finite number of degenerate, periodic, ground states. The appearance of large barriers is owing to the absence of local zero-energy modes that are typical in spin-liquid candidate systems. We establish this by mapping the set of local energy minima states into a tiling with coloured hexagonal tiles. We show that the system exhibits a large number of aperiodic tessellations. The configuration entropy of the local minima is extremely sensitive to boundary conditions, scaling with the boundary length rather than its volume. Characteristics of the resulting state, that is, a rugged energy landscape, where tunnelling from one local minimum to another requires the flipping of a number of spins that grows with system size makes this a distinct state from ordinary spin glass, which we call a spin jam. The low-temperature thermodynamics is also discussed to compare the resulting state with other glassy materials. A tiling problem and the absence of local modes LC states can be conveniently explored as a simple problem of two degrees of freedom: tri-colour (representing the three types of spins for the 120° configuration for the antiferromagnetic linking triangle) and binary sign (representing the parallel (+) or antiparallel (−) direction of each spin within a collinear bipyramid of given colour ( Fig. 1b )) [22] . The triangular network of the bipyramids forces the tri-colour to order long range in a structure as shown by circles in blue, green and red in Fig. 1d . There are 18 possible sign configuration per bipyramid (see Supplementary Fig. 2 ), and the sign degrees of freedom are constrained to have the same sign for each linking triangle that connects each three neighbouring bipyramids (see Supplementary Fig. 3 ) [22] . Spin liquid candidate systems, such as pyrochlore, where any spin configurations with zero spin tetrahedra are ground states have local zero-energy modes, and thus their ground state degeneracy is extensive and scales with the volume. Below, however, we give an entropic argument using a tiling approach to the absence of local zero modes in our model. Absence of such modes greatly enhances the dynamical barrier to transitions between LC states, and facilitates freezing. We map each sign state into a hexagon tile as shown in Fig. 1c . The six corners of the hexagon tile represent the six spins forming the upper and the lower triangles of the bipyramid. The tiles are chosen to have the exact matching and enumeration properties of the sign representation ( Fig. 1b and Supplementary Fig. 4 ), spins on the boundary are associated with black and blue colours according to their sign. The middle spin of the bipyramid does not interact with other bipyramids, and thus we are free to choose the colour of the centre of the hexagon so as to create the simplest patterns that preserve the topology of the network of positive and negative spins on the boundary. Even within the subset of the LC states (sign states), there are numerous ways of covering the entire lattice. With the hexagon representation, the problem of counting the number of sign states in the system becomes a tiling problem (see Supplementary Figs 5 and 6 ). Our tiling problem seems new and bears a remote visual resemblance with a two coloured piecewise Herringbone tiling. To investigate how the degeneracy increases with the size of the system, we first identified numerically all possible sign states with varying the number of columns and rows of bipyramids, and thus varying the size of the system (see Fig. 2a ). As shown in Fig. 2b , for a given column the number of the possible sign states, N , increases with the number of rows in a slower rate than exponentially, which indicates that N does not scale with the volume (area in this quasi-two-dimensional case) of the system. Surprisingly, as shown in the inset, N seems to scale with the number of bipyramids on the boundary, that is, the perimeter of the system. This scaling starkly contrasts with the volume scaling of N of the kagome and pyrochlore systems in which local zero-energy modes exist. This nonextensive scaling may be viewed as a consequence of the absence of local zero-energy modes. Instead, the smallest unit of zero-energy modes scales with the linear dimension of the system, as it involves bipyramids along a line, as shown in Fig. 3a and Supplementary Figs 7 and 8 . 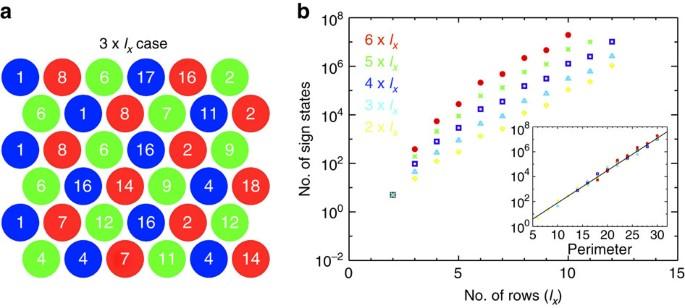Figure 2: Counting the possible collinear bipyramid spin states (sign states). (a) One of the possible sign states constructed numerically for the 3 ×lxbipyramids wherelxis the number of rows. Each circle with a number represents one bipyramid with the sign state assigned by the number. (b) The number of all possible sign states,N, was obtained numerically for different sizes of the system, and plotted in a logarithmic scale as a function oflx. In the inset,Nis plotted as a function of the number of bipyramids on the boundary. The straight line is a guide to eye. Figure 2: Counting the possible collinear bipyramid spin states (sign states). ( a ) One of the possible sign states constructed numerically for the 3 × l x bipyramids where l x is the number of rows. Each circle with a number represents one bipyramid with the sign state assigned by the number. ( b ) The number of all possible sign states, N , was obtained numerically for different sizes of the system, and plotted in a logarithmic scale as a function of l x . In the inset, N is plotted as a function of the number of bipyramids on the boundary. The straight line is a guide to eye. 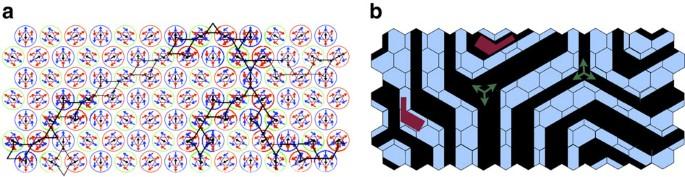Figure 3: An arbitrary collinear bipyramid spin state or a random hexagon tiling. (a) An LC state is shown. At the mean field level, the spins on the black line can rotate collectively without costing any energy, realizing an one-dimensional zero-energy mode. (b) The same state as ina, but shown as a random tiling in the hexagon representation. We have marked to elbows by red to show how lines always switch between thin and thick when changing direction, as long as no junction is involved. A couple of junctions are marked by the green arrows. Full size image Figure 3: An arbitrary collinear bipyramid spin state or a random hexagon tiling. ( a ) An LC state is shown. At the mean field level, the spins on the black line can rotate collectively without costing any energy, realizing an one-dimensional zero-energy mode. ( b ) The same state as in a , but shown as a random tiling in the hexagon representation. We have marked to elbows by red to show how lines always switch between thin and thick when changing direction, as long as no junction is involved. A couple of junctions are marked by the green arrows. Full size image Transfer matrix estimates The nonextensive entropy of the allowed LC states can be examined by using transfer matrix methods. Let us describe the problem as follows. We consider an array of the bipyramids. It may be viewed as alternating two zig-zag columns, which are shifted with respect to each other vertically. We enumerate the possible signs along the zig-zag columns as follows. We consider adding another column in two steps: we first add sites at even levels and then the sites at odd levels as depicted in the Fig. 4 . In this procedure, all the sites in the first stage can be added independently of each other, and after it is completed the second stage shares the same property. 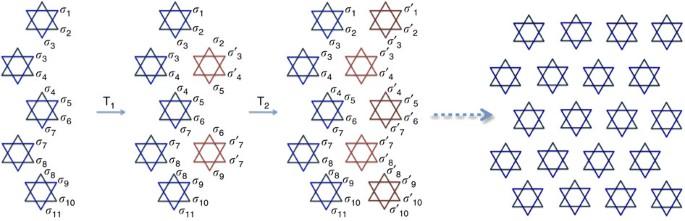Figure 4: Construction of a transfer matrix. Counting of allowed LC configurations can be systematically done using a two step transfer matrix as described above. Given the signs on the right of the first zig-zag column (blue bipyramids on the left), we add an additional column (red), satisfying the ferro-sign constraint in the linking triangles. In the first step, the signsσ1,σ2,σ5,σ6,..σ4n+1,σ4n+2, wherenis an integer, remain unchanged. The sites that might change after the move are of the formσ4n−1,σ4n. A similar addition of a column can then be applied, and the process repeated to cover the lattice. Figure 4: Construction of a transfer matrix. Counting of allowed LC configurations can be systematically done using a two step transfer matrix as described above. Given the signs on the right of the first zig-zag column (blue bipyramids on the left), we add an additional column (red), satisfying the ferro-sign constraint in the linking triangles. In the first step, the signs σ 1 , σ 2 , σ 5 , σ 6 ,.. σ 4 n +1 , σ 4 n +2 , where n is an integer, remain unchanged. The sites that might change after the move are of the form σ 4 n −1 , σ 4 n . A similar addition of a column can then be applied, and the process repeated to cover the lattice. Full size image We are now left with the task of transferring this into a formula. For the bipyramids in the first move, we note that the signs σ 1 , σ 2 , σ 5 , σ 6 ,… and in general σ 4 n +1 , σ 4 n +2 , where n is an integer, remain unchanged. The sites that might change after the move are of the form σ 4 n −1 , σ 4 n . Each such pair only depends on the states of σ 4 n −2 ,.., σ 4 n +1 . Let us denote by m the number of possible sign states with the signs on the left σ 4 n −2 ,.., σ 4 n +1 and sites on the right σ ′ 4 n −1 , σ ′ 4 n , as described in Fig. 4 . We can view this as a linear transformation M with matrix elements: (in particular, m=0 if no move of this type is allowed). For a column of N y bipyramids, there are 2 N y +1 signs on the border that participate in the counting. In the first stage, we can combine all the moves into a larger matrix: Next, we note that the transformation governing the added bipyramids in step 2 is described in the same way, albeit shifted by two sites. In addition, it involves adding boundary bipyramids, which require special counting. We can summarise this as: For N x columns, the number of states may now be computed as , where specify boundary conditions on the left and on the right, respectively. The number of states in a large strip, with N x →∞ scales as λ max ( N y ) N x , where λ max ( N y ) is the largest eigenvalue of the matrix T 2 T 1 . Next, we consider the eigenvalues of T 2 and T 1 separately. These are determined by M . The matrix M is special, and its eigenvalues can be determined analytically. To do so, we first determine the invariant subspaces of this matrix. M is a 16 by 16 matrix, acting on four Ising spins. It turns out more convenient to write it using two double spins, in basis four by assigning: We now find the cycles of the matrix (involving closed subspaces). Explicitly, these consist of the moves (written in basis four) summarised in Table 1 . Interestingly, the six largest eigenvalues are , each doubly degenerate. Here the largest eigenvalue is the golden ratio. As we can bound the norm by , we immediately conclude that the largest eigenvalue of T 1 and of T 2 scale as . From this, we have a rough estimate that the number of states scales at most as . Table 1 Results I of transfer matrix counting. Full size table The two largest eigenvalues of the transfer matrix T 1 T 2 up to 11 rows are summarised in Table 2 . The numerical results show that, at least up to 11 rows, the largest eigenvalue goes down. This means, that for a long enough strip, the number of LC states of 11 rows, will be smaller than, say the number of states of three rows. This behaviour of λ 1 reflects the highly constrained nature of the system, which is consistent with our numerical counting of the allowed LC states shown in Fig. 2 . In the next section, we will put analytical bounds for the entropy of the LC states. Table 2 Results II of transfer matrix counting. Full size table Proving the perimeter scaling of entropy The hexagon representation for the sign state of each bipyramid allows us to establish bounds on the number of LC states, N ( L , V ), for a system of volume V and circumference L . We find that , where K 1 , K 2 are constants. In particular, for V ~ L 2 , we have: , concluding that (up to a possible logarithmic correction) the number of states is extensive in the boundary length. The lower bound is easy to establish: for a given boundary length L , we can construct explicitly a number of states which scales as . One way of doing so is by starting from one of the long-range structures as shown in Fig. 1d,e and Supplementary Fig. 6. These structures support straight quasi one-dimensional modes that change the state of the bipyramid along them. For a square sample of side L , we can put up to L -independent parallel modes of this type, which supplies us with the lower bound. To show the upper bound, we recast the sign states as a tiling problem. We use the hexagonal tiles depicted in Fig. 1c to obtain a representation of the system as a network of lines (see also Supplementary Figs 5 and 6 ). The resultant network may be considered as a fully packed network of rectilinear stripes of alternating colour on a lattice, made of straight lines, π /6 degree turns (‘elbows’) and junctions as shown in Fig. 3b . The network has the following properties (for detailed discussion, see Supplementary Note 1 ): P1. Lines cannot terminate, and P2. There are no closed loops. Property P1 can be verified by inspection of possible termination points, and ruling each of them out. To prove property P2, assume the contrary and consider a closed loop of black colour, inside which there must be loops of smaller and smaller sizes. As the colours alternate, we must have an enclosed simply connected region that is entirely black or entirely blue. As we do not have an entirely blue or entirely black hexagon in our disposal, such a region must be of limited thickness, therefore the inner region must be made of lines with termination points. By property P1, such termination points are not allowed. To proceed, we define a ‘laminar region’ as a region where no junctions are present. Property P3: in a laminar region all lines are locally parallel; moreover, for each of the lines parallel to a chosen reference line (not necessarily a straight one), the thickness at any point along it can be deterministically inferred if the thickness at any other point is known. Property P3 is established by classifying all possible elbow points that do not involve a junction ( Fig. 3b ). Properties P1 and P2 imply that each line must go through the boundary. Property P3 shows that in a laminar region, the thickness degree of freedom of each pattern can be pushed to the boundary; moreover, any elbow must be reflected at two points on the boundary of the sample, a detailed study of these properties shows that for a laminar region we can systematically reconstruct the internal state given the boundary of the region. Next, we consider the presence of junctions and show that N J < L for any network, where N J is the number of junctions. By properties P1 and P2, the network is a graph with the only possible termination points on the boundary, and no closed circles: it is thus a forest (disjoint union of trees), with leaves only on the boundary. An elementary fact of graph theory [27] is that the number of nodes in a full binary tree cannot exceed the number of leaves, therefore N J < L . We can have at most locations for placing junctions in the sample. There is a finite number of possible junction elements. Once the locations and nature of the junctions have been established, the sample excluding the junctions is a laminar region by definition, with effective boundary length proportional to L + N J . Following observation P3, the state is determined by its boundary. Summing over possible numbers of junctions, we have , which yields the aforementioned upper bound. Thus, we have proved that the configurational entropy of the LC states scales with its perimeter rather than its volume. Rugged energy landscape and low-temperature thermodynamics Let us now turn to the energetics of the sign states. Among the myriad of the sign states, there are six long-range ordered states where three types of sign bipyramids are arranged in a structure, one of which is the 1-6-8 state shown in Fig. 1d . Once a sign state is constructed over the entire lattice, the corresponding LC state is constructed by imposing the colour ordering (see Supplementary Fig. 3 ). From the ordered LC states, one can generate noncollinear coplanar bipyramid states (henceforth coplanar states) by collectively rotating each pair of antiparallel spins in each tetrahedron that can be parameterized by three angles (see Supplementary Fig. 9 ) [22] . As listed in Table 3 , the ordered LC states are continuously connected with each other by the collective global rotations through their resulting coplanar states. This rotation can be carried through entirely within the manifold of classical minimum energy spin configurations. On the classical level, such collective motions do not cost any energy, leading to an energy landscape with infinitely large flat bottom formed by collinear and coplanar state and thus, to low-temperature spin liquid behaviours [28] , [29] . Table 3 Connections among the sign states though the global spin rotations. Full size table To investigate what happens when quantum fluctuations are taken into account, we have calculated the energy cost of the quantum fluctuations, within the harmonic (Holstein–Primakoff) approximation around numerous classical spin configurations of minimal energy, with up to 400 bipyramids per sample (involving as many as 2,800 spins). This is done by carrying out numerically a symplectic transformation to diagonalise the resultant bosonic Hamiltonians in real space for each state, without assuming long-range order. It is worth noting that for a material like SCGO, the spin-freezing phenomena occurs at temperatures of a few Kelvin, which are smaller by two orders of magnitude than the typical Heisenberg exchange coupling J , which sets the energy scale for the spin waves. In this regime, thermal fluctuations are negligible. An illustrative example of the procedure is shown in Fig. 5 for 6 × 6 bipyramids with several different LC states as local minima. As the long-range ordered sign state is special, we considered the LC states near the 1-6-8 state that are connected with each other through coplanar states. 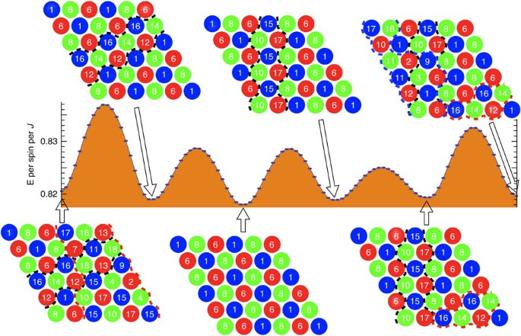Figure 5: Rugged energy landscape induced by quantum fluctuations. The magnetic energy of the quantum fluctuations was calculated for several LC (sign) states near one global minimum. The energy barriers between the minima are composed of the coplanar bipyramid spin states that connect the sign states. Figure 5 shows the results; the degeneracy between the collinear and the coplanar states is lifted, making the LC states local minima and creating energy barriers by the coplanar states. The degeneracy among LC states is also lifted; the sign state has a lower energy than the other sign states, making the long-range ordered state a global minimum and the other LC states local minima. Explicit enumeration shows that there are six possible sign states, giving 36 possible spin states when combined with the six possible colour configurations. Thus, quantum fluctuations lift the mean field ground state degeneracy to form 36 global minima of the long-range ordered LC states and numerous local minima of other LC states, the number of which scales with the perimeter of the system. Note that, as explained above, the selection of the sign states as global minima is an example of a common feature of the order-by-disorder mechanism: that is, the preference of states with the highest symmetry, that is, the smallest magnetic unit cell. Figure 5: Rugged energy landscape induced by quantum fluctuations. The magnetic energy of the quantum fluctuations was calculated for several LC (sign) states near one global minimum. The energy barriers between the minima are composed of the coplanar bipyramid spin states that connect the sign states. Full size image As there are no local spin reorientations that connect between the mean field minima, the dynamical energetic barriers between different states are huge. As a result, on cooling, the system gets trapped in one of the local minima of collinear bipyramids without a long-range order. The spin-freezing explicitly breaks the O(3) invariance of our Heisenberg Hamiltonian. As a result of this symmetry breaking, and the finite spin stiffness for deforming the aperiodic static antiferromagnetic spin texture, its thermodynamics at low temperatures will be governed by low-energy hydrodynamic Halperin–Saslow modes [25] , [30] , [31] (see Supplementary Note 2 for a discussion). Such modes are linearly dispersive and lead to a behaviour for a quasi-two-dimensional system such as ours. Here we make the point that the Halperin–Saslow scenario still holds for the spin jam state, and moreover, is more effective without doping disorder. In conventional spin glasses, where dilute magnetic ions are embedded in a nonmagnetic metal, there is also a linear in T contribution to the specific heat owing to localised two-level systems [32] , which dominates its thermodynamics as observed experimentally [11] . In our system, however, such a linear contribution is negligible at low doping (a point elucidated in ref. 32 ), leading to a behaviour at low temperatures [33] . Another consequence of HS modes is the linear dependence on ω of the imaginary part of the dynamic susceptibility χ ″( ω ) at low frequencies, which contrasts with the frequency-independent χ ″ of the ordinary spin glass [11] . Both features are consistent with the experimentally observed behaviour in SCGO [16] , [33] . While obtaining the freezing temperature precisely in a complex system such as ours is challenging, we can expect the following effect of nonmagnetic doping. For a clean material, the transition temperature to the spin jam state is determined by a competition between the quantum energy cost to flip a set of spins, E SW , and temperature. We therefore expect , where ξ ( T ) is the correlation length in the system. On doping with nonmagnetic impurities, we expect T f to remain unchanged until the typical distance between nonmagnetic impurities becomes comparable to ξ , at which point T f will drop as function of doping concentration. T f behaviour observed in SCGO is consistent with this scenario [21] , [34] . However, in SCGO the Heisenberg coupling J is not uniform, which is manifested in the momentum dependence of elastic neutron scattering [22] . Thus, more work is needed to establish the precise relation to our spin jam state, taking into account specifics of the real material. The concept of a rugged energy landscape was originally proposed to explain freezing phenomenon found in classic spin glass in which dilute magnetic ions in a nonmagnetic metal interact via long-range Ruderman-Kittel-Kasuya-Yosida interactions that change with distance between the magnetic ions and even change in sign [11] . The random magnetic interactions induce frustration, which leads to many states of nearly identical energy and a rugged energy landscape. Since then, it has also been suggested to be responsible for other quenching processes that are ubiquitous in nature, ranging from gelation [35] to metallic glass [8] , to protein folding [36] . In such systems, precise mapping of the complex energy landscape as a function of configurations and thus the microscopic mechanism for the freezing phenomena has been challenging. The triangular network of bipyramids, on the other hand, does not possess the problem of randomness, and thus provides a unique opportunity to microscopically determine the rugged energy landscape and study the mechanism of the spin freezing, as shown in this work. An important ingredient in our treatment was the tiling-based proof that classical local zero modes are absent in the system. We remark that the relevance of tiling as model systems for glassy behaviour has been extensively studied for glasses in the context of kinetically constrained models [13] . As dynamics is usually allowed only when vacancies in the system are present [37] , [38] , a system that is highly packed (or fully packed as in our discussion here) will be ‘stuck’ in a configuration for a very long time. Sub-extensive entropy appears in some kinetically constrained models. For example, the Ising plaquette model on the square lattice exhibits a nonextensive entropy at low temperatures [39] . In this model, glassiness is present on the classical level, and O(3) symmetry is broken on the Hamiltonian level. The system is gapped, rendering trivial low-temperature thermodynamics. This type of models may also be viewed as spin jam models. We would like to stress that our spin jam is induced by quantum fluctuations from clean nearest neighbour Heisenberg interactions, and has non-trivial low-temperature behaviours. Perimeter scaling ground state degeneracy appears in certain compass models as well (for a recent review, see ref. 40 ), where an order-by-disorder mechanism leads to a selection of nematic ground states. In the context of spin liquids, a checkerboard model was studied [41] , where in a valance bond solid phase, bond configurations are stripe-like, and carry entropy that is extensive in boundary length. However, we note that their individual spins have no static moment (in fact, spin configurational entropy is extensive in volume in that model). A valance bond solid state was also suggested on a structurally different but related lattice to ours, a {111} slice of pyrochlore [42] , which has also a volume scaling entropy. A nematic phase of pseudo-spin was explored in S =1 kagome antiferromagnet with a strong single-ion anisotropy [43] , [44] , which is realized without a static spin moment. Finally, we note that similar exotic entropy scaling has been of great interest in other branches of physics, from cosmology, where the entropy of black holes has been argued by Bekenstein and Hawking to scale as the boundary area [45] , [46] , to more recently, in many body quantum mechanical model systems at zero temperature. For example, boundary extensive ground state degeneracy is a feature of some supersymmetric lattice models [47] . A related phenomena is the scaling of entanglement entropy with the boundary area for free scalar fields [46] , that obtains logarithmic corrections when a Fermi surface is present [48] , [49] . In our case, the perimeter scaling entropy is owing to the fact that the local minima of the energy landscape are not separated by local spin rotations (which would typically result in an extensive entropy), but rather are connected with each other by a continuous extended collective rotations of spins, which are sensitive to the states on the boundary. It would be interesting to see if other physical systems possess similar properties. Spin wave calculations To explore the energy landscape generated by quantum fluctuations, we evaluated the spin wave energy contribution to the energy of collinear bipyramid (LC) states and coplanar bipyramid states that are connected by collective spin rotations. The calculations have been done in the framework of the Holstein–Primakoff representation, which we now briefly recall. Consider the Heisenberg Hamiltonian: First, we pick a classical spin configuration that is a local energy minimum, and denote the direction of the spin at position i . In the next step, we replace the spin operator by the Holstein–Primakoff form: where are boson creation/annihilation operators, and are any couple of unit vectors which combine into an orthogonal frame with the classical direction . At this point, to get a tractable theory, the square roots are expanded to lowest order in 1 /S . For a classical spin configuration that is at a classical minimum, this procedure yields in the leading order a quadratic Holstein–Primakoff Hamiltonian H HP in the bosonic operators a i : Where E MF is the mean field energy of the spin configuration. For our semi-classical treatment here, we do not consider higher order terms in 1/ S , responsible for magnon–magnon interactions, as it is well established in practice that for even moderately large spins (such as the S =3/2 for SCGO), quadratic spin wave theory works exceedingly well. For a general spin configuration, the resultant terms appearing in the Hamiltonian are not invariant under translations. However, long-range ordered states have a translational invariant Holstein–Primakoff Hamiltonian H HP . Such states are studied, as usual, by rewriting the Hamiltonian in momentum space. The number of degrees of freedom is then determined simply by the unit size. Bringing the Hamiltonian to a diagonal form, using a Bogolubov transformation yields the form: Where the sum is over the Brillouin zone, and the ‘band’ index α . The contribution of the quadratic terms to the free energy of the system is given by the usual form: where the second term is the thermal corrections and the third term is the zero-point energy. In the case at hand, we assume that J >> k B T , and it follows that the thermal correction is negligible. An example of such a calculation is exhibited in the figure Fig. 6a–d , where different long-range ordered states obtained from 6-1-8 are compared. 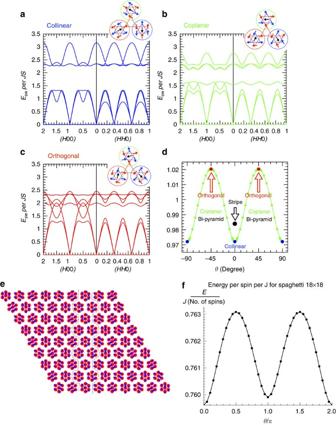Figure 6: Quantum fluctuations lifting classical degeneracy. The magnetic energy of the quantum fluctuations was calculated for several LC (sign) states near one global minimum. The energy barriers between the minima are composed of the coplanar bipyramid spin states that connect the sign states. (a–c) Spin wave dispersions for long-range ordered states obtained from the 6-1-8 state by a global reorientation as described inSupplementary Fig. 9. (d) Integrated spin wave energy as function of rotation angle. Maximum is obtained for orthogonal configurations and minimum for collinear. We also show the energy obtained for the stripe state consisting of alternating rows of 8 and 17 type of sign states (seeSupplementary Fig. 3e). (e) The insertion of a spaghetti mode into an ordered state. The dotted lines in the centre enclose the bipyramids affected by the spaghetti mode. (f) The energy cost of the spaghetti mode as a function of the angle of the rotation of the spaghetti. The energy is divided by the total volume in this graph. Figure 6: Quantum fluctuations lifting classical degeneracy. The magnetic energy of the quantum fluctuations was calculated for several LC (sign) states near one global minimum. The energy barriers between the minima are composed of the coplanar bipyramid spin states that connect the sign states. ( a – c ) Spin wave dispersions for long-range ordered states obtained from the 6-1-8 state by a global reorientation as described in Supplementary Fig. 9 . ( d ) Integrated spin wave energy as function of rotation angle. Maximum is obtained for orthogonal configurations and minimum for collinear. We also show the energy obtained for the stripe state consisting of alternating rows of 8 and 17 type of sign states (see Supplementary Fig. 3e ). ( e ) The insertion of a spaghetti mode into an ordered state. The dotted lines in the centre enclose the bipyramids affected by the spaghetti mode. ( f ) The energy cost of the spaghetti mode as a function of the angle of the rotation of the spaghetti. The energy is divided by the total volume in this graph. Full size image The study of states that are not ordered requires a real space treatment. To diagonalise the Hamiltonian, on a lattice with N=L x L y bipyramids, we get a 7 L x L y quadratic boson Hamiltonian. As H HP is non-interacting in this approximation, the problem is tractable numerically, and amounts to finding a symplectic diagonalisation for a 2*7 L x L y dimensional matrix. To compute the spin wave energies of an arbitrary state of the system, we wrote a programme affecting the symplectic transformations needed to diagonalise the Hamiltonian numerically. We then computed the spin wave energy for the Hamiltonian for various system sizes (as large as 24 × 24 bipyramids, involving a total of 4,032 spins). Fig. 6e shows the insertion of a spaghetti mode into an ordered state, and Fig. 6f shows the energy cost as a function of the angle of the rotation of the spaghetti. How to cite this article: Klich, I. et al. Glassiness and exotic entropy scaling induced by quantum fluctuations in a frustrated magnet. Nat. Commun. 5:3497 doi:10.1038/ncomms4497 (2014).